Polycystin-1 binds Par3/aPKC and controls convergent extension during renal tubular morphogenesis Several organs, including the lungs and kidneys, are formed by epithelial tubes whose proper morphogenesis ensures correct function. This is best exemplified by the kidney, where defective establishment or maintenance of tubular diameter results in polycystic kidney disease, a common genetic disorder. Most polycystic kidney disease cases result from loss-of-function mutations in the PKD1 gene, encoding Polycystin-1, a large receptor of unknown function. Here we demonstrate that PC-1 has an essential role in the establishment of correct tubular diameter during nephron development. Polycystin-1 associates with Par3 favouring the assembly of a pro-polarizing Par3/aPKC complex and it regulates a programme of cell polarity important for oriented cell migration and for a convergent extension-like process during tubular morphogenesis. Par3 inactivation in the developing kidney results in defective convergent extension and tubular morphogenesis, and in renal cyst formation. Our data define Polycystin-1 as central to cell polarization and to epithelial tube morphogenesis and homeostasis. The kidney develops as a result of interactions between the ureteric bud (UB) and the metanephric mesenchyme (MM) [1] . The UB invades the MM and undergoes a series of branchings forming the collecting duct system and ureter of the mature kidney [1] . The UB also induces a condensation and epithelialization of the MM to form comma and S-shaped bodies. The mechanisms responsible for UB branching and MM condensation have been thoroughly studied over the years with important progress being made [1] . By contrast, the mechanisms responsible for the subsequent steps of maturation have been the focus of more recent studies, and many outstanding questions remain [1] . Comma and S-shaped bodies are composed of an immature epithelium with a central lumen, which will undergo a programme of patterning. Both MM- and UB-derived structures undergo a programme of tubular elongation necessary to generate the mature nephron and collecting duct system, respectively [2] . Recent important progress has been made in understanding the mechanisms underlying the elongation process, as well as the establishment and maintenance of tubular diameter [1] , [2] , [3] . This process is achieved by at least two mechanisms. During embryonic development, both the collecting duct and the proximal tubules decrease in diameter. Although cell division is randomly oriented at these stages, tubular elongation involves a process similar to convergent extension (CE) movements, which are known to cause narrowing and elongation of tissues in several systems [1] . It was recently shown that epithelial cells composing the tubules achieve a precise orientation and elongate mediolaterally, in a process resulting in cellular intercalation [3] , [4] . This process depends on the planar cell polarity pathway (PCP) and involves the formation and resolution of rosettes, in a process closely resembling CE [3] . Once this initial phase of morphogenesis is completed (approximately at postnatal day 1 in most collecting ducts in the mouse) and the optimal tubular diameter is reached, further elongation of the tubule is achieved by oriented (proximal–distal) cell division (OCD) [4] , [5] , ensuring elongation, while preserving a correct diameter. Defects in the PCP pathway altering one or both of these processes have been proposed to contribute to cystogenesis [4] , [5] . Defective regulation of tubular diameter is associated with autosomal dominant polycystic kidney disease (PKD), one of the most common inherited disorders [6] . The hallmark of this disease is bilateral renal cyst formation, due to loss-of-function mutations in two genes: PKD1 in 85% of cases or PKD2 in the remaining 15%. Expression of the PKD1 gene is developmentally regulated in the kidneys [7] , suggesting its possible involvement in normal tubular morphogenesis. PKD1 encodes for Polycystin-1 (PC-1), a large plasma membrane receptor of unknown function, with a very large extracellular amino terminus containing protein–protein interaction domains, 11 transmembrane domains and a short intracellular carboxy terminus [7] . PC-1 has been implicated in a number of biological processes [7] , but to date its precise function remains to be defined. The role of the Pkd1 gene in mediating OCD in the tubules of newborn kidneys has been recently investigated and led to controversial results [8] , [9] , whereas the role of PC-1 in tubular morphogenesis and CE during development was not investigated. Here we show that PC-1 is essential for a proper establishment of tubular diameter and mediolateral cell orientation during embryonic renal development in the mouse. PC-1 directly associates with Par3 and favours the association of a Par3/atypical protein kinase C (aPKC) complex in a process likely to be important for oriented cell migration and for renal tubular morphogenesis in the developing kidney. In line with this, we also find that inactivation of the Pard3 gene in the developing kidneys leads to defective CE and to a non-fully penetrant renal cystic phenotype. Defective CE in Pkd1 ΔC/ΔC kidneys To test whether PC-1 is involved in CE during renal development, we analysed a Pkd1 mutant allele previously described by our group, which lacks the last two exons of the gene, resulting in a mutant protein lacking the intracellular C-tail ( Pkd1 ΔC/ΔC ) [10] . These mice die between E.16.5 and E17.5, and display renal cyst formation starting at E15.5 similar to other PKD mice models. The number of cells per cross-section of DBA ( Dolichos biflorus agglutinin)-positive renal tubules in wild-type (wt) kidneys decreased over time from E13.5 to E16.5 ( Fig. 1a,b ), indicating that their diameter decreases (Supplementary Fig. S1). Analysis of Pkd1 ΔC/ΔC mutants showed no significant difference from wt at E13.5 ( Fig. 1a,b ), but a significant defect in tubular narrowing as compared with the wt tubules at later stages (E15.5 and E16.5, Fig. 1a,b,c and Supplementary Fig. S1 ). Staining with Ki67, terminal transferase dUTP nick-end labelling (TUNEL) and cleaved caspase-3 revealed that neither differences in proliferation nor in apoptosis could account for the differences between Pkd1 +/+ and Pkd1 ΔC/ΔC tubules ( Supplementary Fig. S1 ). Conversely, analysis of the morphology of epithelial cells in DBA-positive tubules revealed that the mediolateral orientation normally observed in wt was lost in Pkd1 ΔC/ΔC developing kidneys at E15.5 ( Fig. 1d,e and Supplementary Fig. S1 ). 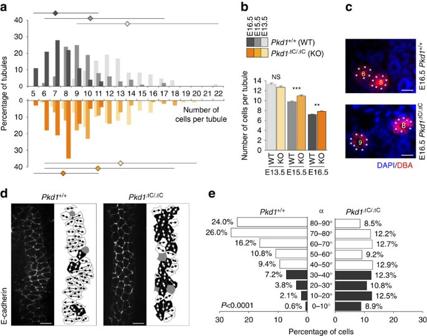Figure 1:Defective tubular narrowing and cellular morphology inPkd1mutants. (a) Histogram of the percentage (yaxis) of DBA-positive tubules with a given number of cells (xaxis) per tubule cross-section at E13.5, E15.5 and E16.5 in wt (top, grey bars) orPkd1ΔC/ΔC(bottom, orange bars) kidneys. The squares and bars on top show the average and the distribution (maximum and minimum numbers), respectively. (b) Graph extrapolated from the data ina. Histograms and bars represent the average and s.e.m. At E13.5,n=183 (wt) andn=182 (KO), and at E15.5 and E16.5,n=200 for both the genotypes, wherenindicates the number of tubules counted. Statistical analysis was carried out by analysis of variance followed by the Bonferroni parameter. NS, nonsignificant; **P<0.01; ***P<0.001. (c) Representative sections of DBA-positive (red) developing tubules at E16.5 ofPkd1+/+orPkd1ΔC/ΔCkidneys. Each cell is labelled with an asterisk and the number of cells per cross-section indicated in the lumen. Scale bar, 20 μm. (d) Confocal images (left panels) and cell outlines (right panels) of frontal sections of E15.5 wt (Pkd1+/+) orPkd1mutant (Pkd1ΔC/ΔC) kidneys stained with an antibody to E-cadherin in DBA-positive sections. Images in the left panels represent sections two frames basal to the aPKC staining, as previously described4. Mediolaterally elongated cells are labelled in white, proximal–distally in black, non-elongated cells in grey. Scale bar, 10 μm. (e) Quantification of the angle of cellular elongation relative to the proximal–distal axis of the tubule forPkd1+/+(left) andPkd1ΔC/ΔC(right). The percentage of cells within each 10° increment is shown. White bars represent cells elongated mediolaterally within a 40°–90° angle. Cells for wt (n=530) and for mutants (n=575) were counted in a minimum of six kidneys from three litters.P<0.0001. Statistical analysis was performed using the Mann–Whitney test. Figure 1: Defective tubular narrowing and cellular morphology in Pkd1 mutants . ( a ) Histogram of the percentage ( y axis) of DBA-positive tubules with a given number of cells ( x axis) per tubule cross-section at E13.5, E15.5 and E16.5 in wt (top, grey bars) or Pkd1 ΔC/ΔC (bottom, orange bars) kidneys. The squares and bars on top show the average and the distribution (maximum and minimum numbers), respectively. ( b ) Graph extrapolated from the data in a . Histograms and bars represent the average and s.e.m. At E13.5, n =183 (wt) and n =182 (KO), and at E15.5 and E16.5, n =200 for both the genotypes, where n indicates the number of tubules counted. Statistical analysis was carried out by analysis of variance followed by the Bonferroni parameter. NS, nonsignificant; ** P <0.01; *** P <0.001. ( c ) Representative sections of DBA-positive (red) developing tubules at E16.5 of Pkd1 +/+ or Pkd1 ΔC/ΔC kidneys. Each cell is labelled with an asterisk and the number of cells per cross-section indicated in the lumen. Scale bar, 20 μm. ( d ) Confocal images (left panels) and cell outlines (right panels) of frontal sections of E15.5 wt ( Pkd1 +/+ ) or Pkd1 mutant ( Pkd1 ΔC/ΔC ) kidneys stained with an antibody to E-cadherin in DBA-positive sections. Images in the left panels represent sections two frames basal to the aPKC staining, as previously described [4] . Mediolaterally elongated cells are labelled in white, proximal–distally in black, non-elongated cells in grey. Scale bar, 10 μm. ( e ) Quantification of the angle of cellular elongation relative to the proximal–distal axis of the tubule for Pkd1 +/+ (left) and Pkd1 ΔC/ΔC (right). The percentage of cells within each 10° increment is shown. White bars represent cells elongated mediolaterally within a 40°–90° angle. Cells for wt ( n =530) and for mutants ( n =575) were counted in a minimum of six kidneys from three litters. P <0.0001. Statistical analysis was performed using the Mann–Whitney test. Full size image PC-1 regulates the front–rear polarity and oriented migration We next aimed at investigating the molecular mechanism underlying this defect. Unfortunately, an appropriate functional assay to study CE or planar polarity in vitro is not available. However, the process of CE is intimately linked to the capability of cells to migrate and orient correctly. Therefore, we used cells derived from Pkd1 +/+ or Pkd1 −/− mice (mouse embryonic fibroblasts, MEFs), in which we have previously reported a defect in migration rates [11] . During our assays, we noticed that in wound-healing assays Pkd1 −/− MEFs took a contorted path to fill the wound, whereas wt cells migrated in a more linear manner ( Fig. 2a,b ). Furthermore, Pkd1 −/− cells failed to relocate their microtubule organizing centre and Golgi in front of their nuclei to generate front–rear polarity as observed in wt cells [12] , [13] ( Fig. 2c ). 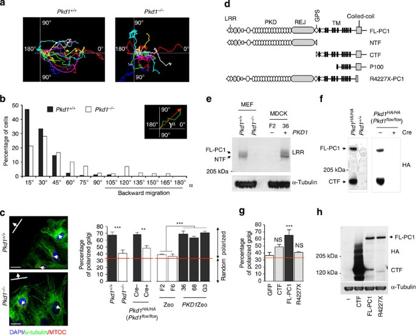Figure 2: PC-1 controls polarized migration. (a) Tracking of cells ofPkd1+/+andPkd1−/−MEFs in 12-h wound-healing time-lapse experiments. Each coloured line is a cell. (b) Scheme and quantification of the experiments ina. The angle of deviationαof each trajectory from a theoretical linear migration (equal to angle 0°) was calculated. Cells (n=102) from nine movies in three independent experiments per cell line. Statistical analysis was performed using the Mann–Whitney test.P<0.0001. (c) Left,Pkd1+/+orPkd1−/−MEFs subject to wound healing followed by IF with an anti-α-tubulin (green), anti-pericentrin (red) and DAPI (blue). Scale bar, 20 μm. Right, quantification of front–rear polarity on three independent MDCKPKD1Zeoclones (36, 68 and G3) and two independent MDCKZeo(F2 and F6), onPkd1+/+orPkd1−/−MEFs orPkd1flox/floxMEFs treated or not with a Cre-recombinase. The red line shows a theoretical random distribution (33%). Statistical analysis was performed using the Student’st-test (for MEFs, left) or analysis of variance (ANOVA; for PKD clones, right) followed by the Bonferroni parameter. **P<0.01; ***P<0.001. Data are means±s.d. and are representative of a minimum of three independent experiments performed in triplicate, in which at least 300 cells were counted. (d) Diagram of PC-1 different isoforms and/or mutant constructs. (e) Immunoblotting of PC-1 in fibroblasts or in MDCKPKD1Zeo(36) and MDCKZeo(F2) using an anti-LRR antibody (7e12, see Methods), detects both the full-length (FL-PC-1, ~520 kDa) and the cleaved, N-terminal fragment (NTF, ~400 kDa). No signal is observed inPkd1−/−cells. (f) Immunoblotting of endogenous tagged PC-1 using an anti-HA detects two bands corresponding to the full-length uncleaved PC-1 (FL-PC-1, ~520 kDa) and the C-terminal fragment (CTF, ~150 kDa). Treatment with a Cre-recombinase causes disappearance of FL-PC-1-HA detection. (g) MDCK type-II cells were transiently transfected with green fluorescent protein alone or along with full-length PC-1 (FL-PC-1), the R4227X or the CTF HA-tagged mutants. After sorting, cells were treated as inc. Data are means±s.d.; Statistical analysis was performed using ANOVA followed by Bonferroni parameter. ***P<0.001, NS, nonsignificant. Figure 2: PC-1 controls polarized migration. ( a ) Tracking of cells of Pkd1 +/+ and Pkd1 −/− MEFs in 12-h wound-healing time-lapse experiments. Each coloured line is a cell. ( b ) Scheme and quantification of the experiments in a . The angle of deviation α of each trajectory from a theoretical linear migration (equal to angle 0°) was calculated. Cells ( n =102) from nine movies in three independent experiments per cell line. Statistical analysis was performed using the Mann–Whitney test. P <0.0001. ( c ) Left, Pkd1 +/+ or Pkd1 −/− MEFs subject to wound healing followed by IF with an anti-α-tubulin (green), anti-pericentrin (red) and DAPI (blue). Scale bar, 20 μm. Right, quantification of front–rear polarity on three independent MDCK PKD1Zeo clones (36, 68 and G3) and two independent MDCK Zeo (F2 and F6), on Pkd1 +/+ or Pkd1 −/− MEFs or Pkd1 flox/flox MEFs treated or not with a Cre-recombinase. The red line shows a theoretical random distribution (33%). Statistical analysis was performed using the Student’s t -test (for MEFs, left) or analysis of variance (ANOVA; for PKD clones, right) followed by the Bonferroni parameter. ** P <0.01; *** P <0.001. Data are means±s.d. and are representative of a minimum of three independent experiments performed in triplicate, in which at least 300 cells were counted. ( d ) Diagram of PC-1 different isoforms and/or mutant constructs. ( e ) Immunoblotting of PC-1 in fibroblasts or in MDCK PKD1Zeo (36) and MDCK Zeo (F2) using an anti-LRR antibody (7e12, see Methods), detects both the full-length (FL-PC-1, ~520 kDa) and the cleaved, N-terminal fragment (NTF, ~400 kDa). No signal is observed in Pkd1 −/− cells. ( f ) Immunoblotting of endogenous tagged PC-1 using an anti-HA detects two bands corresponding to the full-length uncleaved PC-1 (FL-PC-1, ~520 kDa) and the C-terminal fragment (CTF, ~150 kDa). Treatment with a Cre-recombinase causes disappearance of FL-PC-1-HA detection. ( g ) MDCK type-II cells were transiently transfected with green fluorescent protein alone or along with full-length PC-1 (FL-PC-1), the R4227X or the CTF HA-tagged mutants. After sorting, cells were treated as in c . Data are means±s.d. ; Statistical analysis was performed using ANOVA followed by Bonferroni parameter. *** P <0.001, NS, nonsignificant. Full size image Next, we isolated MEFs derived from a mouse model expressing a floxable haemagglutinin (HA)-tagged endogenous PC-1 ( Pkd1 HA/HA or Pkd1 flox/flox interchangeably) [10] . As previously described, HA tags were inserted in-frame into the last exon of the Pkd1 gene, resulting in the expression of HA-tagged endogenous PC-1 (ref. 10 , Fig. 2f ). These lines also carry loxP sites flanking exon 45 and exon 46 (ref. 10 ). Therefore, on treatment with a Cre-recombinase, Pkd1 HA/HA generate the Pkd1 ΔC/ΔC alleles described above, which have lost the protein’s C terminus and its detectability ( Fig. 2c,f ). Importantly, we found that these cells have lost their capability to polarize in wound-healing assays ( Fig. 2c ). Furthermore, a set of Madin–Darby canine kidney, type-II (MDCK type-II) cells overexpressing PC-1 (ref. 14 ) acquired a polarized migratory phenotype as compared with controls ( Fig. 2c ). Finally, transient overexpression of wt FL-PC-1, but not of the patient-derived mutant R4227X (ref. 15 ) or the C-terminal fragment [16] , induced front–rear polarity ( Fig. 2g,h ). Thus, in addition to the previously described capability of PC-1 to regulate cell motility [11] , here we show that PC-1 also regulates the front–rear cell polarity during migration and both the C- and the N-terminal domains are required for this activity. PC-1 binds the Par3/aPKC complex Although the capability of cells to reach appropriate front–rear polarity cannot be considered as an in-vitro assay for CE, the two processes share some molecular factors and mechanisms. One of these is the complex composed of aPKC and the polarity proteins Par3 and Par6, which is very important both for front–rear polarity in mammalian cells and for CE in flies and lower vertebrates [13] , [17] , [18] , [19] , [20] . Therefore, we investigated whether PC-1 could interact or regulate components of the Pars/aPKC complex. To this end, we used MEFs isolated from Pkd1 HA/HA knock-in mice ( Fig. 2f ) [10] . Immunoprecipitation (IP) studies revealed that PC-1 coprecipitates with aPKC, a fraction of which reveal phosphorylation in Thr410 ( Fig. 3a ). In line with this, a kinase-dead mutant of aPKC abrogates the front–rear polarity in MDCK PKD1Zeo cells, suggesting that this kinase is important ( Fig. 3b ), and, in line with published studies, the same mutant abrogated the front–rear polarity in wt MEFs ( Supplementary Fig. S2 ). Notably, endogenous PC-1 coprecipitated Par3 but not Par6 in Pkd1 HA/HA MEFs ( Fig. 3a ), and in reverse IP studies Par3 coprecipitated PC-1 in Pkd1 HA/HA MEFs ( Supplementary Fig. S2 ). To define the domains involved in the interaction, we overexpressed the full-length HA-tagged PC-1 with the 180 kDa or the 100 kDa form of Par3, lacking the aPKC-binding domain ( Fig. 3c ), and found that the overexpressed PC-1 coprecipitated both isoforms ( Fig. 3d ). Furthermore, when the same two constructs were transfected into Pkd1 HA/HA MEF lines, we found that endogenous PC-1 can also interact with both isoforms ( Supplementary Fig. S2 ). Next, we expressed in bacteria the three PDZ domains of Par3, each fused to glutathione S-transferase (GST), and used them in GST pull-down assays along with a histidine-tagged intracellular C-terminal tail of PC-1 (HIS-PC-1-CT) [21] . We found that HIS-PC-1-CT binds to the first two PDZ domains of Par3, but not to the third one ( Fig. 3e ). We conclude that PC-1 C-tail associates directly with Par3 through its first two PDZ domains. These results along with the capability of PC-1 to interact with Par3 lacking the aPKC-binding domain suggest that probably Par3 mediates the interaction between PC-1 and aPKC. 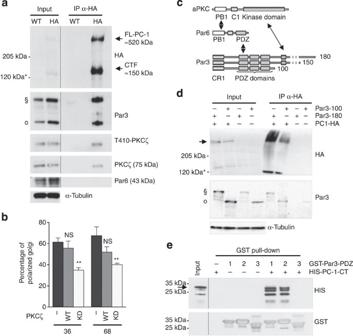Figure 3: PC-1 interacts with the Par3/aPKC complex. (a) MEFs isolated from a mouse model carrying HA-tagged endogenous PC-1 (ref.10) or from littermate embryos (wt) were subject to IP with anti-HA antibodies. Western blotting using anti-HA antibodies revealed the presence of both full-length (arrow, ~520 kDa) as well as cleaved C-terminal fragment (CTF; *, ~150 kDa) isoforms of endogenous, tagged PC-1. Immunoblot analysis of the same IPs using anti-PKCζ and anti-phosphoThr410-PKCζ revealed that PKCζ (78 kDa) interacts with PC-1 in its active form; analysis using anti-Par3 antibodies reveals that PC-1 also coprecipitated with Par3 (180 kDa (§)) and Par3 (100 kDa (°)); analysis using anti-Par6 (43 kDa) antibodies revealed that this molecule is not immunoprecipitated. Blot is representative of multiple independent experiments. (b) Transient transfection of a kinase-dead mutant (KD-PKCζ) or a wt form (WT-PKCζ) in two MDCKPKD1Zeoclones (68 and 36). Data are means±s.d. Statistical analysis was performed using analysis of variance followed by Bonferroni parameter. **P<0.01. NS, nonsignificant. (c) Schematic representation of the aPKC, Par6 and three different isoforms of Par3; arrows indicate the described interacting domains. (d) Hek293T cells were transiently transfected with HA-tagged full-length PC-1 (PC-1-HA) along with the 180 and 100 kDa forms of YFP-Par3, followed by IP with anti-HA antibodies. The blot is representative of two independent experiments. (e) GST-tagged versions of each of the three PDZ domains of Par3 were immobilized on G-sepharose beads, and subsequently incubated with HIS-PC-1-CT. Immunoblotting with anti-GST revealed that equal amounts of GST–PDZ domains of Par3 were immobilized on the beads. Anti-HIS showed that PC-1-CT interacts with the first two PDZ domains, but not with the third. Figure 3: PC-1 interacts with the Par3/aPKC complex. ( a ) MEFs isolated from a mouse model carrying HA-tagged endogenous PC-1 (ref. 10 ) or from littermate embryos (wt) were subject to IP with anti-HA antibodies. Western blotting using anti-HA antibodies revealed the presence of both full-length (arrow, ~520 kDa) as well as cleaved C-terminal fragment (CTF; *, ~150 kDa) isoforms of endogenous, tagged PC-1. Immunoblot analysis of the same IPs using anti-PKCζ and anti-phosphoThr410-PKCζ revealed that PKCζ (78 kDa) interacts with PC-1 in its active form; analysis using anti-Par3 antibodies reveals that PC-1 also coprecipitated with Par3 (180 kDa ( § )) and Par3 (100 kDa (°)); analysis using anti-Par6 (43 kDa) antibodies revealed that this molecule is not immunoprecipitated. Blot is representative of multiple independent experiments. ( b ) Transient transfection of a kinase-dead mutant (KD-PKCζ) or a wt form (WT-PKCζ) in two MDCK PKD1Zeo clones (68 and 36). Data are means±s.d. Statistical analysis was performed using analysis of variance followed by Bonferroni parameter. ** P <0.01. NS, nonsignificant. ( c ) Schematic representation of the aPKC, Par6 and three different isoforms of Par3; arrows indicate the described interacting domains. ( d ) Hek293T cells were transiently transfected with HA-tagged full-length PC-1 (PC-1-HA) along with the 180 and 100 kDa forms of YFP-Par3, followed by IP with anti-HA antibodies. The blot is representative of two independent experiments. ( e ) GST-tagged versions of each of the three PDZ domains of Par3 were immobilized on G-sepharose beads, and subsequently incubated with HIS-PC-1-CT. Immunoblotting with anti-GST revealed that equal amounts of GST–PDZ domains of Par3 were immobilized on the beads. Anti-HIS showed that PC-1-CT interacts with the first two PDZ domains, but not with the third. Full size image PC-1 regulates a balance between Par3/aPKC and Par6/aPKC Next, we looked at the distribution of Par3 in Pkd1 −/− MEFs subject to wound healing and found that these cells fail to properly localize Par3 in distinct patches aligned along the cell–cell contacts, as in wt cells and as previously reported [13] ( Fig. 4a ). Furthermore, IP of aPKC from Pkd1 +/+ and Pkd1 −/− cells revealed that its association with Par3 is reduced, whereas its association with Par6 is enhanced ( Fig. 4b,c ). We hypothesized that changes in the ratio of the Par3 or Par6 bound to aPKC might influence polarized migration. Indeed, overexpression of Par6A was able to displace Par3 from aPKC ( Supplementary Fig. S3 ) and caused an impairment of the front–rear polarity ( Fig. 4d ). Overexpression of Par3 did not have an effect on polarity ( Fig. 4d ), whereas its silencing impaired the front–rear polarity ( Fig. 4d and Supplementary Fig. S3 ). Importantly, overexpression of wt Par6A in Pkd1 HA/HA fibroblasts competes away the association between PC-1 and aPKC in a dose-dependent manner ( Fig. 4e ). Using a Par6 mutant (Par6 K19A ), which lacks the capability to bind aPKC [22] , we found that the interaction between Par6 and aPKC is required for its competing activity ( Fig. 4f ), suggesting that Par6 subtracts aPKC from PC-1/Par3 by binding directly to aPKC. Thus, PC-1 associates with a Par3/aPKC complex (which is in competition with a Par6/aPKC complex) to regulate the front–rear polarity. 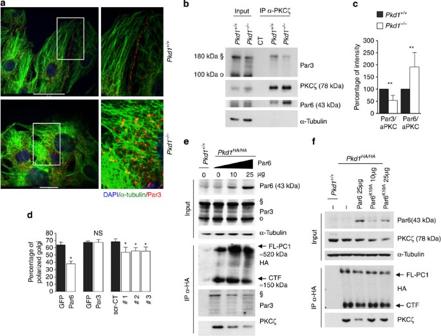Figure 4: PC-1 can influence the ratio of Par3 versus Par6 bound to aPKC. (a) MEF cells were subject to wound, fixed and stained for anti-tubulin (green) and anti-Par3 (red). Scale bars, 20 μm. (b) IP fromPkd1+/+orPkd1−/−MEFs using an anti-PKCζ antibody followed by immunoblotting with an anti-Par3 (180, 150 and 110 kDa) or anti-Par6 (43 kDa) antibody, inPkd1+/+andPkd1−/−MEFs. CT, cell lysate fromPkd1+/+MEFs was incubated in the absence of primary anti-PKC antibody. The blot is representative of seven independent experiments. (c) Quantification of the intensity of bands from seven independent experiments carried out as inb. Data are means±s.e.m. Statistical analysis was performed using analysis of variance (ANOVA) followed by Bonferroni parameter. **P<0.01. (d) Green fluorescent protein (GFP)-positive cells, transfected with GFP, Par6 (GFP, bicistronic vector) or Par3 (180 kDa, YFP-tagged,n=50–120), as well as transfected with three Par3 short interfering RNA (number #1–3,n=600), were analysed for the capability to polarize in wound-healing assays as inFig. 2c. Data are means±s.d., and representative of three independent experiments performed in triplicate. Statistical analysis was performed using ANOVA followed by Bonferroni parameter. *P<0.05, NS, non-statistically significant. (e)Pkd1+/+orPkd1HA/HAMEFs were transfected with increasing amounts of Par6A-expressing constructs, followed by IP with anti-HA beads, followed by western blot analysis with anti-aPKC (78 kDa), anti-Par3 (180 kDa), anti-Par6 (43 kDa) or anti-HA antibodies (full-length PC-1 ~520 kDa and C-terminal fragment (CTF) ~150 kDa). (f) The experiment was performed as ine, except that thePkd1HA/HAMEFs were transfected with Par6 or Par6K19Aconstruct (43 kDa), mutated in the aPKC-binding site22. Figure 4: PC-1 can influence the ratio of Par3 versus Par6 bound to aPKC. ( a ) MEF cells were subject to wound, fixed and stained for anti-tubulin (green) and anti-Par3 (red). Scale bars, 20 μm. ( b ) IP from Pkd1 +/+ or Pkd1 −/− MEFs using an anti-PKCζ antibody followed by immunoblotting with an anti-Par3 (180, 150 and 110 kDa) or anti-Par6 (43 kDa) antibody, in Pkd1 +/+ and Pkd1 −/− MEFs. CT, cell lysate from Pkd1 +/+ MEFs was incubated in the absence of primary anti-PKC antibody. The blot is representative of seven independent experiments. ( c ) Quantification of the intensity of bands from seven independent experiments carried out as in b . Data are means±s.e.m. Statistical analysis was performed using analysis of variance (ANOVA) followed by Bonferroni parameter. ** P <0.01. ( d ) Green fluorescent protein (GFP)-positive cells, transfected with GFP, Par6 (GFP, bicistronic vector) or Par3 (180 kDa, YFP-tagged, n =50–120), as well as transfected with three Par3 short interfering RNA (number #1–3, n =600), were analysed for the capability to polarize in wound-healing assays as in Fig. 2c . Data are means±s.d., and representative of three independent experiments performed in triplicate. Statistical analysis was performed using ANOVA followed by Bonferroni parameter. * P <0.05, NS, non-statistically significant. ( e ) Pkd1 +/+ or Pkd1 HA/HA MEFs were transfected with increasing amounts of Par6A-expressing constructs, followed by IP with anti-HA beads, followed by western blot analysis with anti-aPKC (78 kDa), anti-Par3 (180 kDa), anti-Par6 (43 kDa) or anti-HA antibodies (full-length PC-1 ~520 kDa and C-terminal fragment (CTF) ~150 kDa). ( f ) The experiment was performed as in e , except that the Pkd1 HA/HA MEFs were transfected with Par6 or Par6 K19A construct (43 kDa), mutated in the aPKC-binding site [22] . Full size image PC-1 and Par3 associate in vivo As the Par3/aPKC complex was reported to regulate CE in Drosophila and lower vertebrates [20] , [23] , [24] , we next investigated whether PC-1 interaction with Par3/aPKC could be detected in vivo using our unique murine model of tagged endogenous PC-1 (ref. 10 ). First, we found that the expression levels and cleavage products of PC-1 in the developing kidney in the time window when CE occurs (E13.5 to P1, Fig. 5a–c ) are regulated. Notably, the full-length uncleaved PC-1 levels are maximal in the kidney at E13.5 and progressively decrease during development up to birth; although it is visible in longer exposure times ( Fig. 5c ), the cleaved C-terminal fragment increases progressively and the P100 (ref. 25 ) only appears in the newborn kidneys ( Fig. 5c ). Importantly, the expression pattern of Par3, and specifically the 180 kDa isoform [26] , overlaps with that of full-length PC-1. Second, IP of endogenous HA-PC-1 resulted in coprecipitation of Par3 and aPKC in total embryos at E15.5 ( Fig. 5d ), in the developing kidneys at E17.5 ( Fig. 5e and Supplementary Fig. S2 ) and in P1 newborn kidneys ( Supplementary Fig. S2 ). Finally, we analysed the aPKC complexes and found that IP of aPKC reveals that it preferentially associates with Par3 in Pkd1 +/+ E17.5 kidneys, whereas it preferentially associates with Par6 in E17.5 Pkd1 ΔC/ΔC mutant kidneys ( Fig. 5f,g ). These data are in line with the composition of the complexes observed in cells ( Fig. 4b,c ). As the Pkd1 ΔC/ΔC mutants lack the intracellular C-tail of PC-1, our studies support the notion that this region is essential for PC-1 proper function during renal tubular morphogenesis. 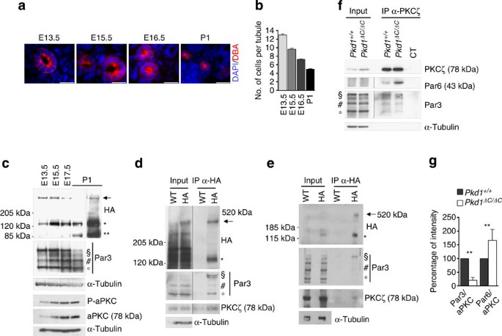Figure 5: PC-1 interacts with and regulates Par3/aPKC in the developing kidneys. (a) Images of DBA-positive tubules at the stages indicated show narrowing of the tubules. Scale bar, 20 μm. (b) Histogram quantifying the process illustrated ina; graphs are average±s.e.m. of the number of cells per tubule cross-section. (c) Western blot analysis on lysates derived from pools of E13.5, E15.5, E17.5 and P1 developing kidneys fromPkd1HA/HAmice, using anti-HA (top panel), anti-Par3 (middle panel) and anti-phosphorylated (T410), or total levels of aPKC antibodies (bottom panel). Representative western blotting of three independent experiments. Arrow, full-length PC-1 (~520 kDa); *, C-terminal fragment (CTF) cleavage product of PC-1 (~150 kDa); **, P100 cleavage product of PC-1 (~100 kDa);§, 180 kDa Par; #, 150 kDa Par3;°, 100 kDa Par3. (d) E15.5 total embryo lysates fromPkd1HA/HA(HA) orPkd1+/+(wt) mice were used to immunoprecipitate PC-1 using anti-HA antibodies, followed by immunoblotting with anti-HA (top), anti-Par3 (middle) or anti-PKCζ antibodies (bottom). Arrow, full-length PC-1 (~520 kDa); *, CTF cleavage product of PC-1 (~150 kDa);§, 180 kDa Par; #, 150 kDa Par3;°, 100 kDa Par3. (e) PC-1 was immunoprecipitated from kidneys ofPkd1HA/HAorPkd1+/+at E17.5 using anti-HA antibodies, followed by immunoblotting with anti-HA, anti- Par3 and anti-aPKC antibodies. Arrow, full-length PC-1 (~520 kDa); *, CTF cleavage product of PC-1 (~150 kDa);§, 180 kDa Par. (f) IP analysis from E16.5Pkd1+/+orPkd1ΔC/ΔCkidneys using an anti-PKCζ antibody followed by immunoblotting with an anti-Par3 or anti-Par6 (43 kDa) antibody. CT, cell lysate fromPkd1+/+embryonic kidneys was incubated in the absence of primary anti-PKC antibody. The blot is representative of three independent experiments. (g) Quantification as means±s.e.m. of the intensity of bands from three independent experiments performed as inf. Statistical analysis was performed using analysis of variance followed by Bonferroni parameter. **P<0.01. Figure 5: PC-1 interacts with and regulates Par3/aPKC in the developing kidneys. ( a ) Images of DBA-positive tubules at the stages indicated show narrowing of the tubules. Scale bar, 20 μm. ( b ) Histogram quantifying the process illustrated in a ; graphs are average±s.e.m. of the number of cells per tubule cross-section. ( c ) Western blot analysis on lysates derived from pools of E13.5, E15.5, E17.5 and P1 developing kidneys from Pkd1 HA/HA mice, using anti-HA (top panel), anti-Par3 (middle panel) and anti-phosphorylated (T410), or total levels of aPKC antibodies (bottom panel). Representative western blotting of three independent experiments. Arrow, full-length PC-1 (~520 kDa); *, C-terminal fragment (CTF) cleavage product of PC-1 (~150 kDa); **, P100 cleavage product of PC-1 (~100 kDa); § , 180 kDa Par; #, 150 kDa Par3; ° , 100 kDa Par3. ( d ) E15.5 total embryo lysates from Pkd1 HA/HA (HA) or Pkd1 +/+ (wt) mice were used to immunoprecipitate PC-1 using anti-HA antibodies, followed by immunoblotting with anti-HA (top), anti-Par3 (middle) or anti-PKCζ antibodies (bottom). Arrow, full-length PC-1 (~520 kDa); *, CTF cleavage product of PC-1 (~150 kDa); § , 180 kDa Par; #, 150 kDa Par3; ° , 100 kDa Par3. ( e ) PC-1 was immunoprecipitated from kidneys of Pkd1 HA/HA or Pkd1 +/+ at E17.5 using anti-HA antibodies, followed by immunoblotting with anti-HA, anti- Par3 and anti-aPKC antibodies. Arrow, full-length PC-1 (~520 kDa); *, CTF cleavage product of PC-1 (~150 kDa); § , 180 kDa Par. ( f ) IP analysis from E16.5 Pkd1 +/+ or Pkd1 ΔC/ΔC kidneys using an anti-PKCζ antibody followed by immunoblotting with an anti-Par3 or anti-Par6 (43 kDa) antibody. CT, cell lysate from Pkd1 +/+ embryonic kidneys was incubated in the absence of primary anti-PKC antibody. The blot is representative of three independent experiments. ( g ) Quantification as means±s.e.m. of the intensity of bands from three independent experiments performed as in f . Statistical analysis was performed using analysis of variance followed by Bonferroni parameter. ** P <0.01. Full size image Defective CE in Par3-mutant kidneys We next reasoned that if direct interaction between PC-1 and Par3 is essential to mediate correct CE and renal tubular narrowing, we would predict that mice mutant for Par3 display a similar defect than Pkd1 mutants. Homozygous deletion of Par3 results in embryonic lethality before E12.5, preventing the analysis of renal development [27] . Thus, we intercrossed a line harbouring a conditional allele for Par3 (ref. 27 ) with a line carrying a Hoxb7:Cre (confining Cre expression in the UB) [28] . Staining of anti-Par3 antibodies confirmed that the protein is lost in a high percentage of cells at E15.5 and at P1 ( Supplementary Fig. S4 ). The resulting mice ( Hoxb7Cre;Par3 flox/− ) displayed a defective number of cells per tubular cross-sections in DBA-positive tubules at E16.5 ( Fig. 6a,b ). Importantly, the Par3 mutants displayed a defective mediolateral orientation of epithelial cells ( Fig. 6c ). A defective number of cells per tubular cross-sections was also observed at P1 ( Fig. 6a,b ), when a few cysts and tubular dilatations were also observed in four out of ten Hoxb7Cre;Par3 flox/− mice ( Fig. 6d ). Importantly, in E15.5 DBA-positive tubules, the rates of cell division were not affected in the Par3 mutants, whereas apoptosis was slightly increased ( Supplementary Fig. S4 ). Furthermore, analysis of markers of apico-basal polarity and tight junctions formation revealed no major defects at this level in the epithelia lacking Par3 ( Fig. 6e and Supplementary Fig. S4 ), in line with previously published studies [26] . We conclude that indeed Par3 is essential for proper CE during renal development in the mouse and that this process is independent of Par3 function in apico-basal polarity, but possibly relies on PCP, as recently demonstrated [5] . 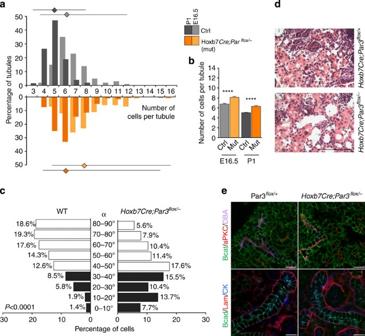Figure 6: Defective CE in Par3 mutants. (a) Histograms showing the distribution of the number of cells per cross-section of tubules as in wt (grey bars,n=100) andHoxb7Cre:Par3flox/−mutant (orange bars,n=100) developing kidneys at E16.5 or P1;nindicates the number of tubules counted. CTRL, controls are eitherHoxb7Cre:Par3flox/+(at P1) orPar3flox/−(at E16.5). (b) Graph extrapolated from the data ina; histograms and bars represent the average and s.e.m. Statistical analysis was performed by analysis of variance (ANOVA) followed by Bonferroni parameter. ****P<0.0001. (c) Quantification of the angle of cellular elongation relative to the proximal–distal axis of the E15.5 tubule for wt orHoxb7Cre:Par3flox/−(right), as inFig. 1e. Four hundred and eighty-three cells for wt and mutants in a minimum of six kidneys from three litters were counted.P<0.0001. Statistical analysis was performed using the Mann–Whitney test. (d) Haematoxylin and eosin staining ofHoxb7Cre:Par3flox/+andHoxb7Cre:Par3flox/−mutant kidneys at P1 show tubular dilatation and small cysts in the Par3 mutants. Scale bar, 100 μm. (e) Sections of control (Par3flox/−, left panel) and mutant (Hoxb7Cre;Par3flox/−, right panel) P1 kidneys stained with antibodies to aPKC (red), β-catenin (green) and the collecting duct maker DBA (purple) in the top panel. In the bottom panel, sections were stained with Laminin (red), E-cadherin (green) and the collecting duct marker cytokeratin (blue). No differences were observed in protein localization/polarity between control and mutant collecting ducts. Scale bar, 20 μm. Figure 6: Defective CE in Par3 mutants. ( a ) Histograms showing the distribution of the number of cells per cross-section of tubules as in wt (grey bars, n =100) and Hoxb7Cre:Par3 flox/− mutant (orange bars, n =100) developing kidneys at E16.5 or P1; n indicates the number of tubules counted. CTRL, controls are either Hoxb7Cre:Par3 flox/+ (at P1) or Par3 flox/− (at E16.5). ( b ) Graph extrapolated from the data in a ; histograms and bars represent the average and s.e.m. Statistical analysis was performed by analysis of variance (ANOVA) followed by Bonferroni parameter. **** P <0.0001. ( c ) Quantification of the angle of cellular elongation relative to the proximal–distal axis of the E15.5 tubule for wt or Hoxb7Cre:Par3 flox/− (right), as in Fig. 1e . Four hundred and eighty-three cells for wt and mutants in a minimum of six kidneys from three litters were counted. P <0.0001. Statistical analysis was performed using the Mann–Whitney test. ( d ) Haematoxylin and eosin staining of Hoxb7Cre:Par3 flox/+ and Hoxb7Cre:Par3 flox/− mutant kidneys at P1 show tubular dilatation and small cysts in the Par3 mutants. Scale bar, 100 μm. ( e ) Sections of control ( Par3 flox/− , left panel) and mutant ( Hoxb7Cre;Par3 flox/− , right panel) P1 kidneys stained with antibodies to aPKC (red), β-catenin (green) and the collecting duct maker DBA (purple) in the top panel. In the bottom panel, sections were stained with Laminin (red), E-cadherin (green) and the collecting duct marker cytokeratin (blue). No differences were observed in protein localization/polarity between control and mutant collecting ducts. Scale bar, 20 μm. Full size image In this study, we have uncovered a critical role for PC-1 in the recently described CE process essential to achieve proper tubular elongation and morphogenesis. In wt developing kidneys, DBA-positive tubules are composed of an average of 13 cells at E13.5 and an average of 7 cells by E16.5. We have shown that in Pkd1 mutant kidneys, DBA-positive tubules fail to undergo this programme of tubular narrowing. Previous studies have shown that the epithelium of the developing nephron divides in a non-oriented manner, but it undergoes mediolateral cellular orientation [4] . As this is a hallmark of tissues undergoing a programme of CE to achieve elongation and narrowing [29] , [30] , this prompted investigators to hypothesize and, subsequently, to demonstrate that the developing nephron is shaped through CE-like movements [3] , [4] . Indeed, cellular intercalation appears to be the mechanism that best explains how epithelial tubules can narrow over time. Here we have shown that the epithelium of DBA-positive tubules lacking functional PC-1 fails to orient mediolaterally, suggesting that PC-1 has an essential role in this process. Our study further uncovers a role for PC-1 in regulation of a programme of cell polarity, enabling cells to properly achieve cellular elongation and front–rear asymmetry during migration in wound-healing assays. We have shown that PC-1 interacts with the aPKC/Par3 (180 kDa) complex and probably regulates it to achieve polarized cell migration. It is interesting to note that PC-1 interacts with both Par3 and aPKC, but not with Par6. Furthermore, the biochemical composition of the aPKC-containing complexes appears to be altered in Pkd1 mutant cells and kidneys. In wt cells, which are able to properly polarize during migration, aPKC preferentially binds to Par3. In contrast, in cells lacking functional PC-1 aPKC appears to preferentially bind to Par6. In addition, overexpression of Par6 is able to compete with Par3 for binding to aPKC and, in line with this, it is able to subtract aPKC from the PC-1/Par3/aPKC complex. This prompted us to hypothesize that Par6 and Par3 might actually compete for binding aPKC. Our data are in line with previous models proposed mostly based on studies in Drosophila , demonstrating that Bazooka (Par3) and Par6 can associate into distinct complexes with different functional roles [31] . Furthermore, a recent study has demonstrated that a competitive binding between Crumbs and Par6 can modulate the exclusion of Par3 from the Par6/aPKC complex, providing further support for a fine-tuned regulation of the so-called ‘Par6/Par3/aPKC complex’ by competitive binding [31] . It is noteworthy that Par3 (180 kDa isoform) and PC-1 appear to follow a similar developmental regulation that parallels the timing of tubular morphogenesis described above. The two proteins are associated in vivo in total embryos and in the developing kidney. We hypothesized that this association might be essential for regulating mediolateral cell orientation and CE during renal tubular morphogenesis. The essential role of the Pars/aPKC complex in regulation of CE downstream of the PCP has been demonstrated in Drosophila melanogaster [20] , [24] , whereas a single study has implicated their role in lower vertebrates [19] . Here we have demonstrated that inactivation of Par3 in the UB of the developing kidney results in defective narrowing of the tubular diameter and defective mediolateral orientation of the epithelia composing these tubules. Thus, our data imply, for the first time, a role of Par3 in CE and tubular morphogenesis in a mammalian system. Although our studies provide important novel insight in the function of PC-1 and its role in renal development, one important question that remains unanswered is whether and how defective CE might result in cyst formation. We show that only ~40% of the Hoxb7Cre:Par3 flox/− mice develop cysts. Thus, defective CE alone might not be sufficient to cause cyst formation and compensatory mechanisms might exist. Similarly, in a previous study, Nishio et al . [8] have shown that defective OCD does not initiate cyst formation in the newborn kidney, as mice mutant for Pkhd1 display defective OCD but not cyst formation. It was proposed that a compensatory mechanism of intercalation might prevent cyst formation in these mice. Thus, one possibility is that neither defects in OCD nor in CE alone are sufficient to initiate cyst formation, but they both might contribute. In summary, in this study we have described a novel role for PC-1 in regulation of a programme of cell polarity, which is important to achieve proper tubular morphogenesis during renal development. Further studies will be required to assess whether this biological function of PC-1 is important for preventing cyst formation and it is relevant for the disease. Antibodies and inhibitors Anti-α-tubulin and anti-flag antibodies were obtained from Sigma (catalogue number 77418-1EA, T5168, T6793 and F1804). Anti phospho-PKCλ/ζ (Thr410/403; catalogue number 9378) was obtained from Cell Signaling. DAPI (catalogue number sc-3598), anti-PKCζ (sc-216/sc-216-G), anti-Par6 (catalogue number sc-14405), anti-PC-1 (catalogue number sc-130554), anti-His (catalogue number sc-8036) and anti-GST (catalogue number sc-495) were obtained from Santa Cruz. Anti-HA from Roche (rat monoclonal catalogue number 13948000). Anti-Par3 was obtained from Millipore (catalogue number 07–330, diluted at 1:300 for immunofluorescence (IF) and at 1:1,000 for western blot). Anti-E-cadherin was obtained from Invitrogen (catalogue number 131900). Anti-Giantin (catalogue number PRB-114C) and anti-pericentrin (catalogue number PRB-432C) were obtained from Covance. Anti-ezrin was obtained from Millipore (07–130, 1:100); anti-occludin from Invitrogen (71–1500, 1:500); and anti-beta-catenin (C7207, 1:500), anti-laminin (l9393, 1:500) and anti-CK from Sigma (C2562, 1:500). Rhodamine conjugated-DBA was obtained from Vector Laboratories (cat RL-1032). All primary antibodies were diluted according to the manufacturer’s instructions unless otherwise stated. HRP-conjugated secondary antibodies (GE Healthcare) were diluted at a 1:7,000 and detection was made with an ECL system (Amersham) Analysis of Pkd1 mutant mice The Pkd1 ΔC mouse model has been previously generated and carries loxP sites flanking the last two exons of the Pkd1 gene (exons 45 and 46) [10] . Timed pregnant mice were obtained by overnight crossing wt or Pkd1 ΔC/+ mice in 100% Bl6/57, and checking for vaginal plugs the next morning. The presence of a vaginal plug was defined as gestational day E0.5 (embryonic day 0.5). All embryos were collected at the defined embryonic stages (between E13.5 and P1 as specified in the legends) and were 50% females and 50% males. The wt and mutant live (based on heart beating) littermate embryos were evaluated from a minimum of three independent litters. All animal care and experimental protocols on the Pkd1 mutants were conducted upon approval of a specific protocol (IACUC-548) by the Institutional Care and Use Ethical Committee at the San Raffaele Scientific Institute. For biochemical studies, we collected and pooled kidneys at day E13.5, 15.5, E17.5 or P1, lysed them with 0.5% triton lysis buffer; IPs were performed as described below for in-vitro studies. Evaluation of tubular diameter in vivo For the evaluation of the number of cells/tubular cross-section, 12 μm sections of E13.5, 15.5, 16.5 or P1 kidneys were stained with the DBA marker and the nuclear marker DAPI. Nuclei of circle-shaped kidney DBA-positive tubules were counted, excluding from analysis the oval-shaped tubules that have values of ovality at the ImageJ software <0.995 (that is, tubules that are not perpendicularly cross-sectioned). We performed two independent experiments for E13.5, E15.5 and E16.5 live (based on heart beating) littermate embryos, counting 100 wt and 100 mutant tubules for each experiment, as well as for P1 wt kidneys. Whenever the phenotype of the embryos was not overt, the analyses were performed in a blinded manner. For the evaluation of circumference and diameter, for round-shaped tubules, a circumference was tracked going through the centre of all the nuclei of the tubular section; the measure of the circumference and of the related Feret’s diameter was quantified by ImageJ software. Evaluation of cellular orientation in vivo For the evaluation of cell elongation and orientation, E15.5 embryos were fixed on in ice-cold methanol, included in 5% low-melting agarose, cut in 100- to 150-μm sections with a vibratome and stained with DBA, anti-E-cadherin, anti-PKCζ antibodies and DAPI. Z -stacks of renal tubules were captured every 1 μm, using UltraView spinning disk confocal microscope (PerkinElmer) with Volocity software. For the evaluation of mediolateral orientation, cell shape was tracked using the automated Magnetic Lasso tool (Photoshop), on E-cadherin staining in sections taken two frames below (basal to) PKC staining. Only cells in the image where E-cadherin staining outlined the entire cell were used for calculations (cells on the edges that had discontinuous E-cadherin staining were not measured). For all other cells, the length (longest axis) to width (shortest axis) ratio were calculated. Only cells for which the ratio was >1.2 were considered elongated. Those that have a lower ratio (between 1 and 1.2) are depicted in grey and are not considered elongated. For all the others, the angle between the longest axis of the cell and the longitudinal axis of the tubule were calculated using ImageJ software [4] . Apoptosis and proliferation in vivo To monitor apoptosis, cryostat kidney sections of 12 μm were stained with TUNEL and the process was carried out using the DeadEnd Fluorometric TUNEL System Kit (Promega), according to the manufacturer’s protocol. Sections were costained for DBA and were used at a dilution of 1/100 (Vector Laboratories). For proliferation, sections were permeabilized in TritonX-100 blocked with PBS–BSA 3% and normal goat serum 10% at room temperature for 1 h, incubated overnight with the antibody anti-Ki67 or anti-Phh3 at 4 °C, washed and incubated with secondary antibodies (Alexa Fluor-conjugated secondary antibodies from Invitrogen–Molecular Probes), and DBA was used at a dilution of 1/100. The ProLong Antifade kit (Invitrogen–Molecular Probes) was used for mounting the samples. Wound-healing assays MDCK type-II and MEF cells were grown on coverslips as high-density monolayers, wounded using a 200-μl pipette tip and allowed to migrate for 3 h (unless otherwise indicated). For IF studies, paraformaldehyde or methanol-fixed cells were washed, permeabilized in PBS/0.5% Triton X-100 and blocked (PBS, 3% BSA). Primary antibody was applied (all antibodies were diluted to 1:100 in blocking and incubated for 1 h at 37 °C) followed by washes and incubation with secondary antibodies (Alexa Fluor-conjugated secondary antibodies from Invitrogen–Molecular Probes). The ProLong Antifade kit (Invitrogen–Molecular Probes) was used for mounting the samples. Digital images of representative fields were captured using a Zeiss Axiophot fluorescence microscope or UltraView spinning disk confocal microscope (PerkinElmer) equipped with a Plan Apochromat 63X/1.4 oil-immersion objective and using the UltraView ERS acquisition software. For time-lapse studies, cells on the wound edge were tracked using the public domain ImageJ programme (developed at the National Institutes of Health and available at http://rsb.info.nih.gov/ij/ ). The rate of unidirectional movement was determined following a minimum of ten different cell trajectories from nine movies of three independent experiments (for a total of 102 cells) and measuring the angle formed by the cell trajectories and the perpendicular movement to the wound edge. Transfection and cell sorting MDCK cells were transiently transfected using Lipofectamine 2000 (Invitrogen). For IP studies, cells were collected at 4 °C in lysis buffer, composed of 150 mM NaCl, 20 mM NaP, 10% glycerol (pH 7.2) supplemented with phosphatase inhibitors (200 mM glycerol phosphate, 200 mM Na orthovanadate and 500 mM Na fluoride), protease inhibitor cocktail (Complete, Roche) and Triton X-100 as indicated. and lysed for 30 min on ice. Nuclei were discarded after centrifugation at 13,200 r.p.m. for 10 min. For HA-tagged PC-1 IP, equal amounts of proteins were incubated overnight at 4 °C with Anti-HA Affinity Matrix (catalogue number 11815016001, Roche); after washes, immunoprecipitates were run on NuPAGE Novex 3–8% TrisAcetate Gel (catalogue number EA0375BOX, Invitrogen). For PKCζ IP studies, equal amount of proteins were incubated in rocking with the primary anti-PKCζ antibody overnight at 4 °C, then G-sepharose beads (catalogue number 17-0618-01, GE Healthcare) were added and incubated 2 h at room temperature. IPs were followed by immunoblotting with the indicated primary antibodies (see above). For cell-sorting experiments, parental MDCK type-II cells were transiently transfected using Lipofectamine 2000 (Invitrogen) according to the manufacturer’s directions by using 12 μg total DNA. For cell sorting, transfections were performed using a construct expressing green fluorescent protein (pEGFP-N1, Clontech) as a marker for cell sorting in combination with PC-1 different constructs (see Fig. 2d ). The following day, cells were analysed by FACS Vantage DIVA sorter (Becton Dickinson). Green fluorescent protein-positive cells were sorted, replated in 60-mm dishes containing coverslips and after 36 h cells were analysed by western blotting or challenged by wound healing followed by IF to nuclei and Golgi/microtubule organizing centre as described. Full images of western blottings are shown in Supplementary Fig. S5 . IP studies and GST pull-down assays For immunoblotting, IP study and GST pull-down assay, lysis buffer composed of 150 mM NaCl, 20 mM NaP, 10% glycerol (pH 7.2) supplemented with phosphatase inhibitors (200 mM glycerol phosphate, 200 mM Na orthovanadate and 500 mM Na fluoride), protease inhibitor cocktail (Complete, Roche) and Triton X-100 as indicated. For GST pull-down assays, the indicated GST-fused PDZ domains of Par3 and HIS-fused C-terminus of PC-1 (aa4132-4303) were expressed in Escherichia coli strain BL21. Bacteria were lysed by sonication in 0.1% Triton X-100 lysis buffer and cleaned by centrifugation. GST-fused protein supernatants were incubated at 4 °C with glutathione beads. Beads were centrifuged, washed and incubated with HIS-fused PC-1 supernatants for 3 h at 4 °C (1:60 in volume of this supernatant was used in immunoblotting as input). After centrifuging and washing the beads, proteins were solubilized in Laemmli buffer and analysed by immunoblotting. Full images of western blottings are shown in Supplementary Fig. S5 . PAR3 silencing Control non-targeting short interfering RNA pool (catalogue number D-001206-13-20) and three short interfering RNA targeting Par3 (Par3#1: 5′-AGACAGACUGGUAGCAGUAUUUU-3′; Par3#2: 5′-GUGAAAUUGAGGUCACGCCUUUU-3′; and Par3#3: 5′-GUGAAAUUGAGGUCACGCCUU-3′), as well as scramble controls were obtained from Thermo Scientific–Dharmacon. To transiently silence Par3, we used Lipofectamine (Invitrogen) transfection, following the manufacturer’s directions. Par3-mutant generation and analysis Hoxb7Cre mice [27] were bred to mice carrying a mutant allele of Pard3 (ref. 26 ). Hoxb7Cre;Par3 +/− males were crossed to females that were homozygous for an allele of Pard3 in which the third coding exon was flanked by loxp sites ( Par3 flox/flox ). Noon of the day of vaginal plugging was considered embryonic day 0.5. Litters (half females and half males) were collected at various timepoints for mutant analysis and genotyped by PCR. For Cre-recombinase, the following primers were used: Hoxb7Cre: forward 5′-GGT CAC GTG GTC AGA AGA GG-3′; Hoxb7Cre: reverse 5′-CTC ATC ACT CGT TGC ATC GA-3′. Presence of Hoxb7Cre results in a 400-bp product. For Par3, the following primers were used: −423iF, 5′-AGG CTA GCC TGG GTG ATT TGA GAC C-3′; −159iR, 5′-TTC CCT GAG GCC TGA CAC TCC AGT C-3′; and +382iF, 5′-GTC TGT GGG GGT TTT GGG AGA GAG G-3′, resulting in products of 371 bp (lox), 292 bp (null) and 265 bp (wt) when resolved on a 3% agarose gel. Mutant embryos ( Hoxb7Cre;Par3 flox/− ) were compared with littermates either with no Cre ( Par3 −/flox ) or no null allele ( Hoxb7cre;Par3 flox/+ ). All animals for these studies were housed, maintained and used according to protocols approved by the Institutional Animal Care and Use Committees at the University of Texas Southwestern Medical Center (animal protocol number 1048-06-01-1). Statistical analysis Student’s t -test or one-way analysis of variance was applied to establish differences between means as indicated in the figure legends. Multiple comparisons were carried out using the Bonferroni parameter. Non-parametric Mann–Whitney test was used for the distribution of the angles of migration ( Fig. 2b and Supplementary Fig. S3 ) and for the distribution of cell orientation in the developing tubules ( Figs 1e and 6c ). How to cite this article: Castelli, M. et al . Polycystin-1 binds Par3/aPKC and controls convergent extension during renal tubular morphogenesis. Nat. Commun. 4:2658 doi: 10.1038/ncomms3658 (2013).